Two-photon interference of weak coherent laser pulses recalled from separate solid-state quantum memories Quantum memories allowing reversible transfer of quantum states between light and matter are central to quantum repeaters, quantum networks and linear optics quantum computing. Significant progress regarding the faithful transfer of quantum information has been reported in recent years. However, none of these demonstrations confirm that the re-emitted photons remain suitable for two-photon interference measurements, such as C-NOT gates and Bell-state measurements, which constitute another key ingredient for all aforementioned applications. Here, using pairs of laser pulses at the single-photon level, we demonstrate two-photon interference and Bell-state measurements after either none, one or both pulses have been reversibly mapped to separate thulium-doped lithium niobate waveguides. As the interference is always near the theoretical maximum, we conclude that our solid-state quantum memories, in addition to faithfully mapping quantum information, also preserve the entire photonic wavefunction. Hence, our memories are generally suitable for future applications of quantum information processing that require two-photon interference. When two indistinguishable single photons impinge on a 50/50 beam splitter (BS) from different input ports, they bunch and leave together by the same output port. This two-photon interference, named the Hong–Ou–Mandel (HOM) effect [1] , is due to destructive interference between the probability amplitudes associated with both input photons being transmitted or both reflected; see Fig. 1 . As no such interference occurs for distinguishable input photons, the interference visibility V provides a convenient way to verify that two photons are indistinguishable in all degrees of freedom, that is, spatial, temporal, spectral and polarization modes. 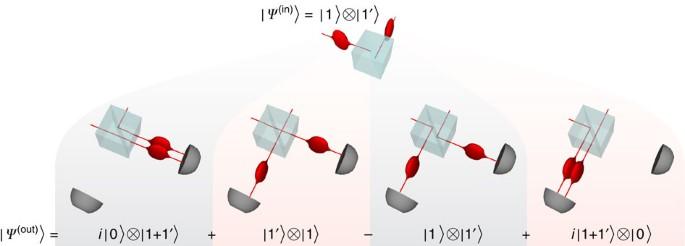Figure 1: Principle of HOM interference. Illustration of HOM interference in the case of single photons at BS input |ψ(in)=|1,1′, where the prime on the latter input indicates the possibility to distinguish that input photon from the other in some degree of freedom, for example, by being polarized orthogonally. The four possible paths of the photons are illustrated, together with their corresponding output states. If the input photons are indistinguishable with respect to all degrees of freedom, we can ignore the primes in the output states and the paths shown in the two central pictures are identical and, because of the different signs, thus cancel. This leaves in the output state |ψ(out)only the possibilities in which photons bunch. For distinguishable photons, for example, having orthogonal polarizations, all paths are distinguishable and all terms remain in |ψ(out). The visibility is defined as Figure 1: Principle of HOM interference. Illustration of HOM interference in the case of single photons at BS input | ψ (in) =|1,1′ , where the prime on the latter input indicates the possibility to distinguish that input photon from the other in some degree of freedom, for example, by being polarized orthogonally. The four possible paths of the photons are illustrated, together with their corresponding output states. If the input photons are indistinguishable with respect to all degrees of freedom, we can ignore the primes in the output states and the paths shown in the two central pictures are identical and, because of the different signs, thus cancel. This leaves in the output state | ψ (out) only the possibilities in which photons bunch. For distinguishable photons, for example, having orthogonal polarizations, all paths are distinguishable and all terms remain in | ψ (out) . Full size image where and denote the rate with which photons are detected in the two output ports in coincidence if the incoming photons are indistinguishable and distinguishable, respectively. Consequently, the HOM effect has been employed to characterize the indistinguishability of photons emitted from a variety of sources, including parametric down-conversion crystals [2] , trapped neutral atoms [3] , [4] , trapped ions [5] , quantum dots [6] , [7] , [8] , organic molecules [9] , nitrogen-vacancy centres in diamond [10] , [11] and atomic vapours [12] , [13] , [14] , [15] , [16] . Further, two-photon interference is at the heart of linear optics Bell-state measurements [17] , and, as such, has already enabled experimental quantum dense coding, quantum teleportation and entanglement swapping [18] . In parallel, recent reports have shown notable progress in mapping light to and from atoms, for example, demonstrating the faithful transfer of quantum information from photons in pure and entangled qubit states [4] , [19] , [20] , [21] , [22] , [23] . However, to date, the possibility to perform Bell-state measurements with photons that have previously been stored in a quantum memory, as required for advanced applications of quantum information processing, has not yet been established. For these measurements to succeed, photons need to remain indistinguishable in all degrees of freedom, which is more restrictive than the faithful recall of quantum information encoded into a single degree of freedom. Indeed, taking into account that photons may or may not have been stored before the measurement, this criterion amounts to the requirement that a quantum memory preserves a photon’s wavefunction during storage. Similar to the case of photon sources, the criterion of indistinguishability is best assessed using HOM interference, provided single-photon detectors are employed. When using single-photon Fock states at the memory inputs, the HOM visibility given in equation (1) theoretically reaches 100% as illustrated in Fig. 1 . However, with phase-randomized laser pulses obeying the Poissonian photon-number statistics, as in our demonstration, the maximally achievable visibility is 50% (ref. 24 ), irrespective of the mean photon number (see Supplementary Note 1 ). Nevertheless, attenuated laser pulses are perfectly suitable for assessing the effect of our quantum memories on the photonic wavefunction. Any reduction of indistinguishability due to storage causes a reduction of visibility, albeit from maximally 50%. Here we demonstrate two-photon interference as well as a Bell-state measurement after either none, one or both weak coherent pulses have been reversibly mapped to separate thulium-doped lithium niobate (Ti:Tm:LiNbO 3 ) waveguides using the atomic frequency comb (AFC) memory protocol [20] , [21] , [25] . The measured interference visibility is always near the theoretical maximum, which verifies that the reversible mapping of the pulses to our solid-state quantum memories preserves the entire photonic wavefunction. Thus, we show that our memories are generally suitable for use in all quantum information processing applications that rely on two-photon interference [26] , [27] . This approach extends the characterization of quantum memories using attenuated laser pulses [28] from assessing the preservation of quantum information during storage to assessing the preservation of the entire wavefunction, and from first- to second-order interference. Experimental overview Our experimental set-up, depicted in Fig. 2 , consists of two cryogenically cooled solid-state quantum memories, elements used to generate optical pulses (that either allow preparing or probing the quantum memories) and devices used to analyse the probe pulses after storage. Light from a 795.43 nm wavelength continuous wave (CW) laser passes through an acousto-optic modulator (AOM) driven by a sinusoidally varying signal. For the memory preparation, we use the AOM’s first negative diffraction order, which is fibre coupled into a phase modulator and, via a BS, two polarization controllers and two micro-electromechanical switches, injected from the back into two Ti:Tm:LiNbO 3 waveguides (labelled A and B ) cooled to 3 K (ref. 29 ). Waveguide A is placed inside a superconducting solenoid. Using a linear frequency-chirping technique [20] , we tailor AFCs with 600 MHz bandwidth and a few tens of MHz peak spacing, depending on the experiment, into the inhomogeneously broadened absorption spectrum of the thulium ions, as shown in Fig. 3 . After 3 ms memory preparation time and 2 ms wait time, we have a 3 ms period during which we store and recall many probe pulses. The 8 ns-long probe pulses with ≈60 MHz Fourier-limited bandwidth are derived from the first positive diffraction order of the AOM output at a repetition rate of 2.5–3 MHz. Each pulse is divided into two spatial modes by a half-wave plate (HWP) followed by a polarizing BS. Pulses in both spatial modes are attenuated by neutral-density filters and coupled into optical fibres and injected from the front into the Ti:Tm:LiNbO 3 waveguides. After exiting the memories (that is, either after storage or direct transmission), the pulses pass quarter- and HWPs used to control their polarizations at the 50/50 BS (HOM-BS) where the two-photon interference occurs. It is noteworthy that, to avoid first-order interference, pulses passing through memory A propagate through a 10 km fibre to delay them with respect to the pulses passing through memory B by more than the laser coherence length, thus randomizing the mutual phase between pulses from the two memories. Finally, pulses are detected by two single-photon detectors (actively quenched silicon avalanche photodiodes) placed at the outputs of the HOM-BS, and coincidence detection events are analysed with a time-to-digital convertor and a computer. 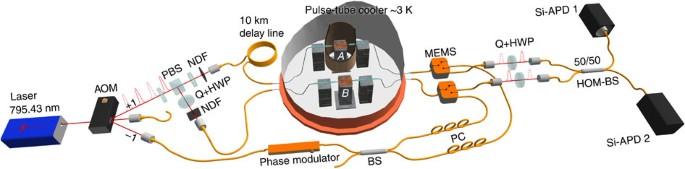Figure 2: Experimental set-up. We employ solid-state quantum memories, more precisely thulium-doped lithium-niobate waveguides, in conjunction with the AFC quantum memory protocol25(see Methods). Using an acousto-optic modulator (AOM) followed by a polarizing beam splitter (PBS) and a neutral-density filter (NDF), we generate weak probe pulses that, after polarization adjustment by a quarter- and a half-wave plate (Q+HWP), are directed to our two memories. After passing through a set of micro electromechanical switches (MEMS), we interfere various combinations of recalled and non-stored (that is, directly transmitted) pulses on a 50/50 BS (HOM-BS) and detect them on silicon avalanche-photodiode (Si-APD)-based detectors as described in the main text. Figure 2: Experimental set-up. We employ solid-state quantum memories, more precisely thulium-doped lithium-niobate waveguides, in conjunction with the AFC quantum memory protocol [25] (see Methods). Using an acousto-optic modulator (AOM) followed by a polarizing beam splitter (PBS) and a neutral-density filter (NDF), we generate weak probe pulses that, after polarization adjustment by a quarter- and a half-wave plate (Q+HWP), are directed to our two memories. After passing through a set of micro electromechanical switches (MEMS), we interfere various combinations of recalled and non-stored (that is, directly transmitted) pulses on a 50/50 BS (HOM-BS) and detect them on silicon avalanche-photodiode (Si-APD)-based detectors as described in the main text. 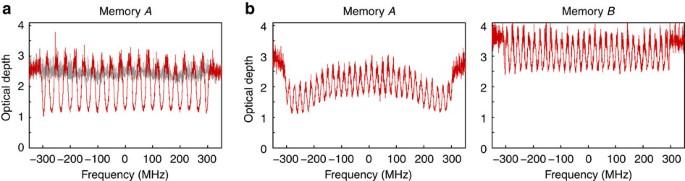Figure 3: Absorption spectra of quantum memories. Measured absorption spectra of AFCs prepared in Ti:Tm:LiNbO3waveguides using frequency-selective optical pumping for the (a) single-memory and (b) two-memory configurations (red traces). The light grey trace inashows the optical depth when the memory is inactive, that is, no AFC is prepared. The AFC bandwidths are set to 600 MHz, which is much wider than that of the stored pulses (about 60 MHz). The AFC peak spacing inais Δ=33 MHz and inbΔ=20 MHz, yielding storage times of 1/Δ=30 and 50 ns, respectively. In the depicted AFC for the single-memory configuration (a), a 133 Gauss magnetic field is applied along thecaxis of crystalA—located inside the magnet solenoid (seeFig. 2)—causing the excited and ground states to split into two long-lived nuclear Zeeman sublevels. The resulting splitting difference of Δ/2≈17 MHz gives the optimal memory efficiency. In the two-memory configuration (b) it is important to note that memoryBis located outside the solenoid and thus experiences a different field than memoryA. To obtain recall efficiencies that are reasonably similar, at the expense of being non-optimal, we set the magnetic field at memoryAto 900 G (see Methods). Full size image Figure 3: Absorption spectra of quantum memories. Measured absorption spectra of AFCs prepared in Ti:Tm:LiNbO 3 waveguides using frequency-selective optical pumping for the ( a ) single-memory and ( b ) two-memory configurations (red traces). The light grey trace in a shows the optical depth when the memory is inactive, that is, no AFC is prepared. The AFC bandwidths are set to 600 MHz, which is much wider than that of the stored pulses (about 60 MHz). The AFC peak spacing in a is Δ=33 MHz and in b Δ=20 MHz, yielding storage times of 1/Δ=30 and 50 ns, respectively. In the depicted AFC for the single-memory configuration ( a ), a 133 Gauss magnetic field is applied along the c axis of crystal A —located inside the magnet solenoid (see Fig. 2 )—causing the excited and ground states to split into two long-lived nuclear Zeeman sublevels. The resulting splitting difference of Δ/2≈17 MHz gives the optimal memory efficiency. In the two-memory configuration ( b ) it is important to note that memory B is located outside the solenoid and thus experiences a different field than memory A . To obtain recall efficiencies that are reasonably similar, at the expense of being non-optimal, we set the magnetic field at memory A to 900 G (see Methods). Full size image HOM measurements after single-photon-level storage We first deactivate both quantum memories (see Methods) to examine the interference between directly transmitted pulses, thereby establishing a reference visibility for our experimental set-up. We set the mean photon number per pulse before the memories to 0.6, that is, to the single-photon level. Using the wave plates, we rotate the polarizations of the pulses at the two HOM-BS inputs to be parallel (indistinguishable) or orthogonal (distinguishable) and in both cases record the coincidence detection rates of the detectors at the HOM-BS outputs. Employing equation (1), we find a visibility of (47.9±3.1)%. Subsequently, we activate memory A while keeping memory B off and adjust the timing of the pulse preparation so as to interfere a recalled pulse from the active memory with a directly transmitted pulse from the inactive memory (see Methods). Pulses are stored for 30 ns in memory A prepared with the AFC shown in Fig. 3a , and the mean photon number per pulse at the quantum memory input is 0.6. Taking the limited storage efficiency of ≈1.5% and coupling loss into account, this results in 3.4 × 10 −4 photons per pulse at the HOM-BS inputs. As before, changing the pulse polarizations from mutually parallel to orthogonal, we find V =(47.7±5.4)%, which equals our reference value within the measurement uncertainties. As the final step, we activate both memories to test the feasibility of two-photon interference in a quantum-repeater scenario. We note that in a real-world implementation, memories belonging to different network nodes are not necessarily identical in terms of material properties and environment. This is captured by our set-up where the two Ti:Tm:LiNbO 3 waveguides feature different optical depths and experience different magnetic fields (see Fig. 3b and Methods). To balance the ensuing difference in memory efficiency, we set the mean photon number per pulse before the less efficient and more efficient memories to 4.6 and 0.6, respectively, so that, as before, the mean photon numbers are 3.4 × 10 −4 at both HOM-BS inputs. With the storage time of both memories set to 30 ns, we find V =(47.2±3.4)% in excellent agreement with the values from the previous measurements. The consistently high visibilities, compiled in the first column of Table 1 , hence confirm that our storage devices do not introduce any degradation of photon indistinguishability during the reversible mapping process, and that two-photon interference is feasible with photons recalled from separate quantum memories, even if the memories are not identical. Table 1 Experimental two-photon interference visibilities for different degrees of freedom. Full size table HOM measurements after storage of few-photon pulses We now investigate in greater detail the change in coincidence count rates as photons gradually change from being mutually indistinguishable to completely distinguishable with respect to each degree of freedom accessible for change in single-mode fibres, that is, polarization, temporal and spectral modes (see Methods). To acquire data more efficiently, we increase the mean number of photons per pulse at the memory input to between 10 and 50 (referred to as few-photon-level measurements). However, the mean photon number at the HOM-BS remains below one. Example data plots are shown in Fig. 4 , whereas the complete set of plots is supplied in Supplementary Figs S1–S3 . 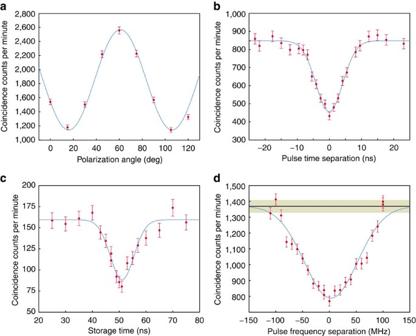Figure 4: Examples of measured HOM interference. HOM interference plot examples for one or two active memory configurations. (a) Varying mutual polarization difference with one active memory and 30 ns storage time. (b) Varying temporal overlap by changing timing of pulse generation with two active memories and 50 ns storage time. (c) Varying temporal overlap by changing storage time of one active quantum memory from 25 to 75 ns. (d) Varying spectral overlap for one active quantum memory and 50 ns storage time. Owing to the limited frequency tuning range of our AOM, we determine a reference level by additionally making the pulse polarizations orthogonal. The resulting count rate is shown with the black line and error band in dark yellow. All error bars are calculated—assuming the Poissonian counting statistics—as the square-root of the total counts. Some additional scattering is because of intensity fluctuations at the HOM-BS inputs, which cannot be normalized away using the counts from the individual detectors owing to the manifestation of the HOM interference in these counts (seeSupplementary Note 5). The data in (a) are fitted to a sinus function. The data inb–dare fitted to a Gaussian function. The acquisition time per data point is 60 s ina,b,dand 120 s inc. Figure 4: Examples of measured HOM interference. HOM interference plot examples for one or two active memory configurations. ( a ) Varying mutual polarization difference with one active memory and 30 ns storage time. ( b ) Varying temporal overlap by changing timing of pulse generation with two active memories and 50 ns storage time. ( c ) Varying temporal overlap by changing storage time of one active quantum memory from 25 to 75 ns. ( d ) Varying spectral overlap for one active quantum memory and 50 ns storage time. Owing to the limited frequency tuning range of our AOM, we determine a reference level by additionally making the pulse polarizations orthogonal. The resulting count rate is shown with the black line and error band in dark yellow. All error bars are calculated—assuming the Poissonian counting statistics—as the square-root of the total counts. Some additional scattering is because of intensity fluctuations at the HOM-BS inputs, which cannot be normalized away using the counts from the individual detectors owing to the manifestation of the HOM interference in these counts (see Supplementary Note 5 ). The data in ( a ) are fitted to a sinus function. The data in b – d are fitted to a Gaussian function. The acquisition time per data point is 60 s in a , b , d and 120 s in c . Full size image In Fig. 4a , we show the coincidence count rates as a function of the polarization of the recalled pulse for the case of one active memory. The visibilities for all configurations (that is, zero, one or two active memories) extracted from fits to the experimental data are listed in column 2 of Table 1 . They are—as in the case of single-photon-level inputs—equal to within the experimental uncertainty. Next, in Fig. 4b , we depict the coincidence count rates as a function of the temporal overlap (adjusted by the timing of the pulse generation) for the two-memory configuration. Column 3 of Table 1 shows the visibilities extracted from Gaussian fits to the data, reflecting the temporal profiles of the probe pulses, for all configurations. Within experimental uncertainty, they are equal to each other. Alternatively, in the single-memory configuration, we also change the temporal mode overlap by adjusting the storage time of the pulse mapped to the quantum memory. Again the measured visibility of V =(44.4±6.9)% (see Fig. 4c ) is close to the theoretical maximum. Finally, we vary the frequency difference between the two pulses to witness two-photon interference with respect to spectral distinguishability. For this measurement, we consider only the configurations in which neither, or a single memory is active. In both cases, the visibilities, listed in the last column of Table 1 , are around 43%. Although this is below the visibilities found previously, for reasons discussed in the Supplementary Note 2 , the key observation is that the quantum memory does not affect the visibility. We have now demonstrated several experiments that consistently yield high two-photon interference visibilities; however, we wish to point out that the two-photon interference visibility can be substantially reduced by imperfect preparation or operation of our quantum memory. This is further discussed in the Supplementary Note 3 . Bell-state measurement As stated in the introduction, Bell-state measurements (BSM) with photonic qubits recalled from separate quantum memories are key ingredients for future applications of quantum communication. To demonstrate this important element, we consider the asymmetric (and arguably least favourable) configuration in which only one of the qubits is stored and recalled. Appropriately driving the AOM in Fig. 2 , we alternately prepare the states | Ψ a and | Ψ b , which describe time-bin qubits [18] of the form , where e and l , respectively, label photons in early- or late-temporal modes, which are separated by 25 ns. The parameter θ k determines the relative amplitude of and ϕ k the relative phase between the two temporal modes composing the time-bin qubit for k =a,b. The qubits are directed to the memories of which only one is activated. The mean photon number of the qubit that is stored is set to 0.6, yielding a mean photon number of both qubits at the HOM-BS input of 6.7 × 10 −4 . We ensure to overlap pulses encoding the states | Ψ a and | Ψ b at the HOM-BS and count coincidence detections that correspond to a projection onto the Bell state. This projection occurs if the two detectors click with 25 ns time difference [18] . The count rate of the projection can be generalized for any given states of two incoming time-bin qubits as (see Supplementary Note 4 ) where we assume equal mean photon numbers μ at the two HOM-BS inputs. As | ψ − is antisymmetric with respect to any basis, the count rate is expected to reach a minimum value if the two input pulses are prepared in equal states ( Ψ a | Ψ b =1), and a maximum value if prepared in orthogonal states ( Ψ a | Ψ b =0). Accordingly, we define an error rate that quantifies the deviation of the minimum count rate from its ideal value of zero: We now consider two important cases for which we will compute the error rates both in theory and from our experiment. For qubits with ϕ a = ϕ b =0 (that is, encoded onto the xz -plane of the Bloch sphere), we are interested in the rate for the case in which the input qubits are parallel ( θ a = θ b ) and for the case in which the input qubit states are orthogonal ( θ a = θ b − π ). Specifically, when we prepare two qubits (one at each input of the HOM-BS) in state | e , or two qubits in state | l , we expect from the expression given in the equation (2). The count rate for observing a projection onto | ψ − increases as we change θ a (or θ b ), and reaches a maximum if one qubit is in state | e and the other one in | l . Hence, using the expression for the error rate from equation (3), we find , where the superscript (att) indicates that this result applies to attenuated laser pulses. We now turn to measuring the coincidence rates for all combinations of | e and | l input states, thus extracting and , using 0.6 photons per qubit at the memory input. More precisely, we prepare the input qubit state to measure and then to measure . Subsequently, we prepare the input qubit state to measure and then to measure . These yield the average values and , from which we compute the experimental error rate , which is near the theoretical value of . Next, we consider the case in which two input qubits are in equal superpositions of early and late bins, and , that is on the xy -plane of the Bloch sphere ( θ a = θ b = π /2). Using equation (2), we find that the | ψ − Bell-state projection count rate is smallest—but non-zero—when ϕ a – ϕ b =0, that is, the qubit states are parallel, and largest when the phases differ by π , that is, the qubit states are orthogonal. Inserting the respective values for and into equation (3) results in an expected error rate of . Using again 0.6 photons per qubit, we measure the coincidence counts for ϕ a – ϕ b =0 and π , giving us and , respectively. From these we get an experimental error rate of , which is slightly above the theoretical bound. This indicates that either the measurement suffers from imperfections such as detector noise, or the modes at the HOM-BS are not completely indistinguishable, which, in turn, could be due to imperfectly generated qubit states or imperfect storage of the qubit in the quantum memory. In the following, we will use the measured error rates to asses our quantum memory and thus make the most conservative assumption that the entire differences between the expected and measured values for the error rates are due to the memory fidelity being less than one. Assessing our quantum memory using Bell-state measurements As a first step, we derive lower bounds for the error rates when the best-known classical storage strategy is applied, and then compare it to the outcomes of our Bell-state measurements. To accommodate this scenario, we suppose that the memory performs the following operation | ψ ψ |→ F | ψ ψ |+(1– F )| |, where F denotes the fidelity of the stored state and | is the state orthogonal to the input state | ψ . For storing a photon in an unknown qubit state, the fidelity is bounded from above by F CM =0.667 when using a classical memory [30] , whereas for a quantum memory the upper bound is F QM =1. The former bound strictly only applies to the storage of single-photon states, whereas, for coherent states, the bound is higher. Indeed, the best classical storage approach is optimized with respect to the mean number of photons per qubit and derives additional information about an input state by measuring individual photons from signals containing multiple photons in different bases. Further, if the quantum memory features limited efficiency, then the best classical memory would selectively discard signals containing one (or few) photon(s) and measure only signals containing large numbers of photons. This would allow keeping the total recall efficiency unaffected while maximizing the fidelity. The adjusted bound, , has been derived in refs 4 , 31 . Given our mean photon number per qubit of 0.6 together with 0.3% system efficiency (1.5% memory and 20% waveguide coupling efficiencies), we compute . The fidelity of the memory operation modifies the Bell-state measurement count rates as , and likewise for . This allows us to express the error rate expected after imperfect storage of one of the qubits partaking in the Bell-state measurement: where the count rates and are those expected without the memory. After simple algebra using equation (2) and equation (4), we find that for the qubits encoded in the e / l basis, and, using , yields a lower bound of with a classical memory. Hence, our experimentally observed value of clearly violates the bound. In the +/− basis, we derive , which, in the case of an optimized classical memory, yields the lower bound . Our measured value of is again below the classical limit. We can also reverse the equations and estimate our memory’s fidelity based on the measured error rates. In this case, inserting and into the appropriate expressions in the previous paragraph, we deduce the values and . The measured estimates of the memory fidelity and in the two bases are equal to within the experimental error and well above the upper bound for an optimized classical memory. Although we do not use single-photon sources for the experiments reported here, it is interesting to determine how well our results measure up to those that could have been obtained if single-photon sources had been employed. For this, one can simply compute the count rate for the projection onto | ψ − for arbitrary two input qubits encoded into single photons (see Supplementary Note 4 ). We find that for any two parallel input qubit states ( θ a = θ b and ϕ a = ϕ b ) we get . Therefore, irrespective of the projection count rate for orthogonal input qubit states, the expected error rate is always e (sing) =0, where ‘sing’ identifies this value as belonging to the single-photon case. Gauging the effect of storing one of the single photons partaking in the Bell-state measurement in a memory is thus independent of the basis and, using equation (4), we derive e (sing) =1– F and specifically compute the bound e (sing,CM) =0.333. We recognize that the two values and obtained experimentally are both well below e (sing,CM) . This means that even with a single-photon source at ones disposal, the error rates that we measured could not have been attained with a classical memory. In this study, we demonstrate two-photon interference of weak coherent laser pulses recalled from separate AFC-based waveguide quantum memories. Our measurement results show that the two-photon interference visibility stays near the theoretical maximum of 50% regardless of whether none, one or both pulses have been recalled from our quantum memories. In addition, we demonstrate for the first time a Bell-state projection measurement with one of the two partaking qubits having been reversibly mapped to a quantum memory—a key element for advanced applications of quantum information processing. Our results show that solid-state AFC quantum memories are suitable for two-photon interference experiments, even in the general case of storing the two photons an unequal number of times. Further, we analyse quantum and classical bounds of the storage fidelity for Bell-state measurements with weak laser pulses and assess the quantum nature of our storage device by comparing our experimental results to the derived theoretical bounds. This approach follows the practice of employing attenuated laser pulses to characterize quantum memories [4] , [28] , [31] , however, extending it from assessing the preservation of quantum information encoded in a single degree of freedom to assessing the preservation of all degrees of freedom of the photonic wavefunction. As long as the dark count rate is low, our memories’ efficiencies do not affect the measured error rates as these are based on post-selected coincidence detection events. Thus, our results pertain to the numerous applications, such as quantum repeaters, which incorporate post-selection. Given these results, our quantum memories may soon be used as synchronization devices in multi-photon experiments. This will require an improvement of the system efficiency [32] and implementation of multi-mode storage supplemented by read-out on demand. The latter requirement can be achieved by storing photons occupying different temporal modes and adjusting the recall time of the photons [33] . Alternatively, it can be achieved by simultaneously storing photons in different spectral modes and selectively recalling photons in certain frequency modes (N.S., manuscript in preparation), which does not require adjustable storage time. This will allow increasing the number of photons that can be harnessed simultaneously for quantum information processing or fundamental tests beyond the current limit of eight [34] . A further goal is to develop workable quantum repeaters or, more generally, quantum networks, for which longer storage times are additionally needed. Depending on the required value, which may range from a 100 ms (ref. 35 ) to seconds [26] , this may be achieved by storing quantum information in optical coherence, or it may require mapping of optical coherence onto spin states [25] . Preparation and properties of our quantum memories The fabrication of the Ti:Tm:LiNbO 3 waveguides and spectroscopic properties of Tm atoms in this material have been reported in ref. 29 . The two waveguides are fabricated identically but differ in terms of overall length, yielding optical depths of 2.5 for memory A and 3.6 for memory B . To prepare an AFC memory, we perform frequency-selective optical pumping on the inhomogeneously broadened transition of Tm at 795.43 nm wavelength. This process is determined by two factors, namely the spectrum of the pumping light, averaged over many pumping cycles, and the level structure of Ti:Tm:LiNbO 3 . As detailed in ref. 20 , the optical pumping is achieved by chirping the laser frequency while periodically modulating its intensity. Resonant atoms are excited and subsequently decay to a long-lived shelving state, yielding a spectral hole at the excitation wavelength. Hence, repeating this process a sufficiently long time using pump light with (time-averaged) periodic spectrum results in periodic persistent spectral holes that form the troughs of the AFC. The atoms that are not excited by the pump light remain in the ground state and form the peaks of the AFC. Once the AFC is prepared, an incident photon is mapped onto a collective excitation of thulium ions and subsequently re-emitted after a pre-set storage time given by t =1/ Δ , where Δ is the comb tooth spacing [25] . As the spectrum of the optical pumping light controls Δ , it allows one to set the storage (delay) time. In our storage devices, Ti:Tm:LiNbO 3 crystals, the ground and shelving states are formed by the two nuclear Zeeman-levels that become non-degenerate with the application of a magnetic field along the C 3 axis of the crystals. To optimally prepare an AFC, we adjust the magnetic field such that the difference of the ground and excited-level splittings matches the frequency separation between the AFC’s troughs and peaks. The AFC in memory A for the single-memory configuration is shown in Fig. 3a . It is noteworthy that as memory A is located at the centre of the set-up’s solenoid while memory B is outside the solenoid (see Fig. 2 ), it is not possible to apply the same magnetic field across the two crystals. Hence, we cannot, in the two-memory configuration, generate the optimal-level splittings for both memories simultaneously. Instead, we apply a magnetic field that provides a reasonable balance in recall efficiencies but is not optimal for either memory. This is reflected by the different optical-depth profiles and reduced contrasts of the AFCs shown in red in Fig. 3b . Memory operation A quantum memory is said to be activated when we configure the micro-electromechanical switches to allow the optical pumping light to reach the memory during the preparation stage, and thus tailor an AFC into the inhomogeneously broadened absorption spectrum of thulium (see Fig. 2 ). If the optical pumping is blocked, the memory is said to be deactivated and light entering the waveguide merely experiences constant attenuation over its entire spectrum. In all cases, we adjust the mean photon number at the memory inputs so that mean photon numbers are equal at the HOM-BS inputs. This is required for achieving maximum visibility with attenuated laser pulses (see Supplementary Note 1 ). Changing degrees of freedom The polarization degree is easily adjusted using the free-space half- and quarter-wave plates set at each HOM-BS input. For our measurements, we rotate the HWP in steps of either 45° or 7.5°. The temporal separation δ t between a pulse arriving at one of the HOM-BS inputs and the next pulse in the train arriving at the other input can be expressed as δ t ={ nl / c }mod δ t r , where n is the refractive index of the fibres, l ≈10 km is the path-length difference for pulses interacting with memory A and B , and δ t r is the repetition period of the pulse train from the AOM, which is set in the range of 350–400 ns. As we can change δ t r with 10 ps precision, we can tune δ t on the ns scale. For the storage time scan, the recall efficiency decreases with storage time because of decoherence. Hence, we balance the mean photon number per pulse for stored and transmitted pulses for each storage time. Finally, to change the spectral overlap of the pulses input to the HOM-BS, we can utilize that these pulses were generated at different times in the AOM and thus we can choose their carrier frequencies independently. We interchangeably drive the AOM by frequencies ν a and ν b and thus create two interlaced trains of pulses with different frequencies. By adjusting the pulse timing, we can ensure that the pulses overlapped at the HOM-BS belong to different trains and thus have a spectral overlap given by δ ν = ν a – ν b . Owing to the limited bandwidth of the AOM, we are only able to scan δ ν by 100 MHz, which, when compared with the 60 MHz pulse bandwidth, is not quite sufficient to make the pulses completely distinguishable. To achieve complete distinguishability, we supplement with a measurement using orthogonal polarizations at the inputs (see Supplementary Note 2 ). Preparing states for Bell-state measurement For the Bell-state projection measurement, we interchangeably prepare time-bin qubits in either | e or | l , or in and by setting the relative phase and intensity of the AOM drive signal. Adjusting the timing of the pulse preparation, we ensure that qubits in different states overlap at the HOM-BS. How to cite this article: Jin, J. et al. Two-photon interference of weak coherent laser pulses recalled from separate solid-state quantum memories. Nat. Commun. 4:2386 doi: 10.1038/ncomms3386 (2013).